Constitutive and ligand-induced EGFR signalling triggers distinct and mutually exclusive downstream signalling networks Epidermal growth factor receptor (EGFR) overexpression plays an important oncogenic role in cancer. Regular EGFR protein levels are increased in cancer cells and the receptor then becomes constitutively active. However, downstream signals generated by constitutively activated EGFR are unknown. Here we report that the overexpressed EGFR oscillates between two distinct and mutually exclusive modes of signalling. Constitutive or non-canonical EGFR signalling activates the transcription factor IRF3 leading to expression of IFI27, IFIT1 and TRAIL. Ligand-mediated activation of EGFR switches off IRF3-dependent transcription, activates canonical extracellular signal-regulated kinase (ERK) and Akt signals, and confers sensitivity to chemotherapy and virus-induced cell death. Mechanistically, the distinct downstream signals result from a switch of EGFR-associated proteins. EGFR constitutively complexes with IRF3 and TBK1 leading to TBK1 and IRF3 phosphorylation. Addition of epidermal growth factor dissociates TBK1, IRF3 and EGFR leading to a loss of IRF3 activity, Shc-EGFR association and ERK activation. Finally, we provide evidence for non-canonical EGFR signalling in glioblastoma. Increased activation of the epidermal growth factor receptor (EGFR) signalling pathway is common in cancer and may correlate with tumour development and/or progression. Common mechanisms underlying aberrant EGFR signalling include increased expression of the EGFR, overproduction of ligands, EGFR mutation and constitutive activation [1] , [2] . It is estimated that one-third of all epithelial cancers express high levels of EGFR [3] . EGFR overexpression may occur with or without EGFR gene amplification in cancer. EGFR gene amplification and increased EGFR expression are detected in 40–50% of glioblastoma (GBM), the most common malignant adult brain tumour [4] , [5] . As the EGFR is commonly overexpressed in cancer, it has generated intense interest for a role in the pathogenesis of tumours and as a target for treatment [6] . EGFR wild-type (EGFRwt) expression can transform cells and generate tumours, either alone or in conjunction with loss of tumour suppressors [7] , [8] , [9] . Furthermore, overexpression of the EGFR ligand TGF-α can induce cancer in transgenic mice [10] , [11] . Increased EGFR activity may result in cancer cell proliferation, inhibition of apoptosis, motility, invasion and metastasis, and angiogenesis [12] , [13] , [14] . The EGFR is composed of a single extracellular ligand-binding domain, a transmembrane domain and a cytoplasmic domain containing a conserved protein tyrosine core [15] , [16] . Ligand binding leads to conformation changes in the extracellular domain of the EGFR resulting in EGFR activation and downstream signalling [17] . The formation of asymmetric dimers of kinase domains has been reported to be a key step in EGFR activation and the EGFR is allosterically activated in an asymmetric dimer [18] , [19] . Activation of the EGFR results in formation of specific signalling complexes that culminate in gene transcription and a biological response [20] . Recent studies have shown that dimerization occurs even in the absence of ligand, particularly when the EGFR is overexpressed and may be restricted to subsets of dimers [21] . In addition, overexpressed EGFR may dimerize and become tyrosine phosphorylated in the absence of ligand [22] , [23] . However, it has remained unclear whether this ligand-independent EGFR activation results in activation of downstream signals. IRF3 is a transcription factor that plays a key role in antiviral innate immunity. TBK1 and IKKε have been identified as kinases essential for phosphorylation of IRF3 in response to viral infection or dsRNA [24] , [25] . Phosphorylation of IRF3 resulting in its activation, nuclear translocation and induction of gene transcription. In this study, we show that overexpression of the EGFR in cancer cells results in a bimodal programme of signal transduction and identify a pathway that is activated by constitutive EGFR signalling in cancer. In the absence of ligand, the EGFR signals constitutively and activates the transcription factor IRF3, resulting in transcription of genes involved in the antiviral and innate immune response. When epidermal growth factor (EGF) is added, the activation of IRF3 is lost, and the EGFR now activates canonical downstream signalling pathways such as extracellular signal-regulated kinase (ERK) and Akt. Thus, ligand-independent and -dependent signalling pathways appear to be mutually exclusive. The EGFR constitutively activates IRF3 by recruiting IRF3 and its kinase TBK1 to the EGFR, with resultant phosphorylation and activation of IRF3 that results in transcription of target genes. Addition of EGF results in a loss of the ternary complex between EGFR, IRF3 and TBK1, loss of IRF3 phosphorylation and abrogation of the transcriptional activity of IRF3. The biological effect of EGFR-mediated IRF3 activation appears to be protection from virus-induced cell death and this effect may confer an advantage during the clonal evolution of tumours. Concomitant with the termination of IRF3 activity with ligand, there is activation of known oncogenic EGFR pathways such as ERK and Akt and induction of known early genes such as EGR1 and EGR2 . Thus, the availability of ligand acts as a switch to turn off IRF3-dependent signalling and trigger known oncogenic signalling pathways such as ERK and Akt. Interestingly, ligand-mediated activation of EGFR renders it more sensitive to chemotherapy, suggesting that the presence of EGFR ligand within the tumour may influence response to treatment. Finally, we present evidence demonstrating that constitutive or non-canonical EGFR signalling is active in human cancer. Constitutive and ligand-induced EGFR signalling is distinct Unless specified otherwise, we use the term EGFR for EGFR wild-type (EGFRwt) in this study. Previous studies have indicated that when the EGFR is overexpressed it becomes tyrosine phosphorylated and constitutively activated [21] , [22] . However, the downstream signals generated by constitutively activated EGFR are unknown. In a previous study, we found that conditional expression of EGFRwt in response to tetracycline resulted in transcription of a significant number of genes even without exogenous EGF [26] . In this previous study, we used microarray analysis and compared gene expression profiles of U251 cells overexpressing EGFRwt and compared the results to vector-transfected U251 cells. We found that 93 genes were upregulated by EGFR overexpression in the absence of exogenous EGF and 55 genes were downregulated. Sixty-six genes were upregulated only when EGF was added and eight genes were downregulated [26] . 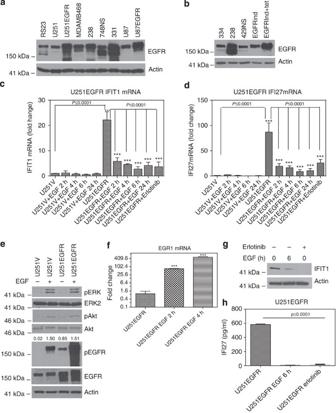Figure 1: Constitutive EGFR signalling. (a,b) Western blot showing EGFR levels in various cell lines, lysates prepared directly from frozen resected GBM tumour tissue (RS23, 238, 331, 334) and primary neurosphere cultures derived from GBMs (748NS and 429NS). The lower-molecular-weight bands identified by the EGFR antibody may be partially degraded EGFR. Cells were cultured in serum-free DMEM overnight for experimentsc–h. The EGF concentration used was 50 ng ml−1. (c) Quantitative real-time PCR examining IFIT1 mRNA levels in U251EGFR cells and in empty vector-transfected U251V cells. In U251EGFR cells, IFIT1 level is high in the absence of EGF and diminishes in response to EGF exposure (P<0.0001). (d) The same experiment examining IFI27 mRNA shows similar results (P<0.0001). (e) U251V or U251EGFR cells were treated with EGF for 15 min followed by preparation of lysates and western blot with the indicated antibodies. Densitometry was performed for pEGFR/EGFR and the values are shown. (f) An experiment examining mRNA levels of EGR1 in U251EGFR cells. In contradistinction to IFIT1 and IFI27, EGR1 is low in the absence of EGF and increase when cells are exposed to EGF (P<0.001). (g) Protein levels of IFIT1 were examined in U251EGFR cells by western blot. There is a decrease in IFIT1 levels with the addition of EGF or when cells are exposed to Erlotinib (10 μM, overnight). (h) ELISA for IFI27 levels in U251EGFR cells shows a high level of IFI27 in the absence of EGF. When EGF is added IFI27 levels are decreased. Exposing cells to Erlotinib also results in a decrease in IFI27 levels. Error bars represent the means±standard deviations of three independent experiments. Data were analysed by one-way ANOVA followed by Tukey’s multiple comparison test. *P≤0.05, **P≤0.01, ***P≤0.001. These include a number of genes involved in interferon signalling shown in Supplementary Table 1 in our previous study [26] . Furthermore, a 90-min exposure to EGF did not result in a further increase in expression of these genes [26] . However, autocrine and paracrine loops are common in glioma cells [27] , [28] and whether such loops were responsible for what appeared to be constitutive EGFR signalling was not investigated in that study. In the current study, we examine constitutive and ligand-induced EGFR signalling in detail using constitutive as well as conditional overexpression of EGFR, at levels similar to that seen in human cancer. Thus, we used U251MG or U87MG cells constitutively overexpressing EGFR (U251EGFR, U87EGFR), and U251MG cells conditionally overexpressing EGFR in response to tetracycline (U251EGFRind). EGFR signalling was also examined in primary GBM neurospheres cultured in stem cell medium and in MDAMB468 breast cancer cells that spontaneously express a high level of EGFR. The EGFR levels in these lines and in actual tumours are shown in Fig. 1a,b . Figure 1: Constitutive EGFR signalling. ( a , b ) Western blot showing EGFR levels in various cell lines, lysates prepared directly from frozen resected GBM tumour tissue (RS23, 238, 331, 334) and primary neurosphere cultures derived from GBMs (748NS and 429NS). The lower-molecular-weight bands identified by the EGFR antibody may be partially degraded EGFR. Cells were cultured in serum-free DMEM overnight for experiments c – h . The EGF concentration used was 50 ng ml −1 . ( c ) Quantitative real-time PCR examining IFIT1 mRNA levels in U251EGFR cells and in empty vector-transfected U251V cells. In U251EGFR cells, IFIT1 level is high in the absence of EGF and diminishes in response to EGF exposure ( P <0.0001). ( d ) The same experiment examining IFI27 mRNA shows similar results ( P <0.0001). ( e ) U251V or U251EGFR cells were treated with EGF for 15 min followed by preparation of lysates and western blot with the indicated antibodies. Densitometry was performed for pEGFR/EGFR and the values are shown. ( f ) An experiment examining mRNA levels of EGR1 in U251EGFR cells. In contradistinction to IFIT1 and IFI27, EGR1 is low in the absence of EGF and increase when cells are exposed to EGF ( P <0.001). ( g ) Protein levels of IFIT1 were examined in U251EGFR cells by western blot. There is a decrease in IFIT1 levels with the addition of EGF or when cells are exposed to Erlotinib (10 μM, overnight). ( h ) ELISA for IFI27 levels in U251EGFR cells shows a high level of IFI27 in the absence of EGF. When EGF is added IFI27 levels are decreased. Exposing cells to Erlotinib also results in a decrease in IFI27 levels. Error bars represent the means±standard deviations of three independent experiments. Data were analysed by one-way ANOVA followed by Tukey’s multiple comparison test. * P ≤0.05, ** P ≤0.01, *** P ≤0.001. Full size image To further examine constitutive EGFR signalling, we looked at EGFR-induced expression of IFIT1 and IFI27 expression by quantitative real-time PCR. These two genes were selected for their robust expression in response to EGFR overexpression and lack of further increase in response to EGF in our previous study. A high level of IFIT1 and IFI27 expression was observed in U251EGFR cells compared with vector-transfected cells confirming that IFIT1 and IFI27 expression is driven by EGFR ( Fig. 1c,d ). Surprisingly, addition of EGF to cells abrogated EGFR-induced expression of IFIT1 and IFI27 ( Fig. 1c,d ) arguing against an autocrine mechanism for expression of these genes. In addition, inhibition of EGFR kinase activity with Erlotinib results in a block of IFIT1 and IFI27 induction, indicating that these genes are induced by EGFR activity ( Fig. 1c,d ). Importantly, although increasing EGFR expression in multiple cell lines results in tyrosine phosphorylation of the EGFR, it does not result in ERK or Akt activation unless EGF is added ( Fig. 1e , and Supplementary Fig. 1a,b ), suggesting that constitutive and ligand-induced signalling networks are distinct. EGFR overexpression leads to constitutive tyrosine phosphorylation of multiple tyrosine residues in the EGFR tail as shown in Supplementary Fig. 1c . Although the level of EGFR phosphorylation detected in EGFR-overexpressing cells in the absence of ligand is low compared with ligand-stimulated cells, it is clearly detectable and is detected only in EGFR-overexpressing cells ( Supplementary Fig. 1d,e ). Ligand-induced activation of EGFR is known to induce rapid expression of a number of genes. We confirmed that concomitant with the downregulation of IFIT1 and IFI27, the genes EGR1 and EGR2 are rapidly upregulated by EGF in U251EGFR cells ( Fig. 1f and Supplementary Fig. 2a ). EGF-mediated downregulation of IFIT1 and IFI27 was confirmed at a protein level by western blot and ELISA, respectively ( Fig. 1g,h ). To rigorously exclude an autocrine mechanism for constitutive EGFR-mediated induction of IFIT1 and IFI27, we examined the effect of Cetuximab, which blocks ligand binding to the EGFR. Cetuximab failed to inhibit EGFR-mediated IFIT1 and IFI27 upregulation while effectively blocking EGF-mediated tyrosine phosphorylation of the EGFR, arguing against an autocrine mechanism ( Fig. 2a,b and Supplementary Fig. 2b ). Next, conditional expression of EGFRvIII, a non-ligand-binding EGFR mutant found in GBM, upregulates IFIT1 and IFI27 in U251MG cells ( Fig. 2c,d and Supplementary Fig. 2c ), excluding an intracellular mechanism of autocrine stimulation. A kinase-inactive EGFR mutant failed to upregulate IFIT1 and IFI27 ( Fig. 2e,f and Supplementary Fig. 2d ). Thus, multiple lines of evidence suggest that EGFR generates a distinct signalling programme in the absence of ligand. Similar results were detected in the breast cancer cell line MDAMB468 cells ( Supplementary Fig. 3a–d ) and in U251EGFRind cells, in which EGFR is conditionally expressed in response to tetracycline ( Supplementary Fig. 4a,b ), in U87EGFR cells ( Supplementary Fig. 4c–e ) and in glioma-initiating cells derived from a GBM and cultured as neurospheres (429NS) shown in Fig. 1b and Supplementary Fig. 5a,b . In all these cell lines, increased EGFR expression induces the upregulation of IFIT1 and IFI27 in the absence of ligand. When EGF is added, the induction of these genes is lost. These data also indicate that constitutive EGFR signalling is detected only in cells with increased EGFR expression and may be specific to cancer, a disease in which EGFR is frequently overexpressed. We also examined the expression of a third gene, TRAIL and again found a similar pattern with upregulation of TRAIL in the absence of EGF and downregulation when EGF is added ( Supplementary Fig. 5c–e ). 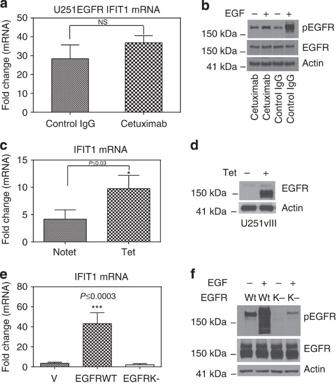Figure 2: Constitutive EGFR signalling requires EGFR kinase activity but not ligand. (a) Cetuximab fails to inhibit EGFR-mediated induction of IFIT1 mRNA as detected by real-time quantitative PCR. Cells were incubated overnight with either control IgG or Cetuximab (100 μg ml−1). (b) Cetuximab effectively blocks EGF-induced tyrosine phosphorylation of EGFR. Cells were incubated overnight with Cetuximab or control IgG followed by exposure to EGF for 15 min followed by western blot with pEGFR antibody. (c) U251 cells conditionally expressing the mutant EGFRvIII in response to tetracycline were incubated with tetracycline (or no tetracycline) for 24 h followed by RNA extraction and quantitative PCR (qPCR) for IFIT1. (d) Western blot showing expression of EGFRvIII in U251 cells following tetracycline exposure. EGFRvIII is truncated and migrates faster on electrophoresis gels compared with endogenous EGFRwt. (e) U251 cells were transfected with EGFRwt, a kinase-inactive EGFR mutant, or empty vector followed by extraction of RNA and qPCR for IFIT1. (f) Expression of EGFRwt results in increased tyrosine phosphorylation of EGFR, which is further and substantially increased by EGF stimulation, whereas the EGFR kinase mutant fails to become tyrosine phosphorylated in response to EGF (an increase in tyrosine phosphorylation of the small amount of endogenous EGFRwt is seen). Cells were serum starved and cultured in serum-free DMEM overnight for all experiments. The EGF concentration used was 50 ng ml−1. Error bars represent the means±standard deviations of three independent experiments. Data were analysed by one-way ANOVA followed by Tukey’s multiple comparison test. *P≤0.05, **P≤0.01, ***P≤0.001. Figure 2: Constitutive EGFR signalling requires EGFR kinase activity but not ligand. ( a ) Cetuximab fails to inhibit EGFR-mediated induction of IFIT1 mRNA as detected by real-time quantitative PCR. Cells were incubated overnight with either control IgG or Cetuximab (100 μg ml −1 ). ( b ) Cetuximab effectively blocks EGF-induced tyrosine phosphorylation of EGFR. Cells were incubated overnight with Cetuximab or control IgG followed by exposure to EGF for 15 min followed by western blot with pEGFR antibody. ( c ) U251 cells conditionally expressing the mutant EGFRvIII in response to tetracycline were incubated with tetracycline (or no tetracycline) for 24 h followed by RNA extraction and quantitative PCR (qPCR) for IFIT1. ( d ) Western blot showing expression of EGFRvIII in U251 cells following tetracycline exposure. EGFRvIII is truncated and migrates faster on electrophoresis gels compared with endogenous EGFRwt. ( e ) U251 cells were transfected with EGFRwt, a kinase-inactive EGFR mutant, or empty vector followed by extraction of RNA and qPCR for IFIT1. ( f ) Expression of EGFRwt results in increased tyrosine phosphorylation of EGFR, which is further and substantially increased by EGF stimulation, whereas the EGFR kinase mutant fails to become tyrosine phosphorylated in response to EGF (an increase in tyrosine phosphorylation of the small amount of endogenous EGFRwt is seen). Cells were serum starved and cultured in serum-free DMEM overnight for all experiments. The EGF concentration used was 50 ng ml −1 . Error bars represent the means±standard deviations of three independent experiments. Data were analysed by one-way ANOVA followed by Tukey’s multiple comparison test. * P ≤0.05, ** P ≤0.01, *** P ≤0.001. Full size image EGFR-mediated regulation of IFIT1 and IFI27 was also confirmed at a protein level in MDAMB468 cells and U87EGFR cells ( Supplementary Figs 3c,d,4e ). IFIT1 levels are high in the absence of ligand and downregulated with EGF, consistent with the quantitative PCR findings. Cetuximab blocked the EGF-mediated downregulation of IFIT1 ( Supplementary Fig. 4f ). Constitutive EGFR signalling is mediated by IRF3 activation Many of the genes induced by constitutive EGFR signalling are known IRF3 target genes. For example, IFIT1, IFI27 and TRAIL are all known to be expressed via transcriptional activation of IRF3 (refs 25 , 29 ). We silenced IRF3 using short interfering RNA (siRNA) and compared constitutive EGFR-induced expression of IFIT1 and IFI27 in U251EGFR cells. Silencing of IRF3 blocked constitutive EGFR-induced expression of these genes compared with control (scrambled) siRNA-transfected cells ( Fig. 3a,b ). A similar result was found in U87EGFR cells ( Supplementary Fig. 6a–c ). Furthermore, re-expression of IRF3 following IRF3 knockdown restored EGFR-induced expression of IFIT1 and IFI27, arguing against a nonspecific siRNA effect and supporting a specific role for IRF3 ( Fig. 3d–f ). These experiments suggest that IRF3 is required for EGFR-mediated upregulation of IFIT1 and IFI27. 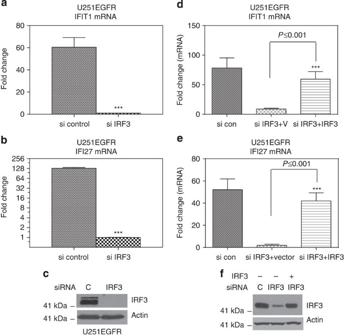Figure 3: IRF3 is required for constitutive EGFR signalling. (a,b) U251EGFR cells were transfected with control (scrambled) siRNA or with siRNA directed against IRF3 followed by quantitative real-time PCR for IFIT1 or IFI27. The mRNA levels for both genes are decreased when IRF3 is silenced compared with control siRNA (si Con; unpairedt-test,P<0.0001). (c) Silencing of IRF3 by western blot. Ind,e, U251EGFR cells were transfected with IRF3 siRNA (for 72 h) followed by re-expression of IRF3 (or empty vector) and extraction of RNA after 48 h for quantitative PCR for IFIT1 and IFI27. (f) Western blot showing silencing of IRF3 and re-expression in silenced cells. Error bars represent the means±standard deviations of three independent experiments. Data were analysed by one-way ANOVA followed by Tukey’s multiple comparison test. *P: ≤0.05, **P≤0.01, ***P≤0.001. Figure 3: IRF3 is required for constitutive EGFR signalling. ( a , b ) U251EGFR cells were transfected with control (scrambled) siRNA or with siRNA directed against IRF3 followed by quantitative real-time PCR for IFIT1 or IFI27. The mRNA levels for both genes are decreased when IRF3 is silenced compared with control siRNA (si Con; unpaired t -test, P <0.0001). ( c ) Silencing of IRF3 by western blot. In d , e , U251EGFR cells were transfected with IRF3 siRNA (for 72 h) followed by re-expression of IRF3 (or empty vector) and extraction of RNA after 48 h for quantitative PCR for IFIT1 and IFI27. ( f ) Western blot showing silencing of IRF3 and re-expression in silenced cells. Error bars represent the means±standard deviations of three independent experiments. Data were analysed by one-way ANOVA followed by Tukey’s multiple comparison test. * P : ≤0.05, ** P ≤0.01, *** P ≤0.001. Full size image Constitutive EGFR signalling results in IRF3 activation IRF3 is a key transcription factor involved in antiviral responses and is activated by stimuli such as double-stranded RNA and Toll-like receptor (TLR) signalling [29] . IRF3 is known to bind to the interferon-sensitive response element (ISRE). To investigate whether constitutive EGFR signalling results in transcriptional activation of IRF3, we conducted a reporter assay with a synthetic ISRE-LUC reporter as well as an IFI27 ISRE-LUC reporter. EGFR overexpression and constitutive EGFR signalling results in transcriptional activation of IRF3 in U251EGFR, U87EGFR and MDAMB468 cells ( Fig. 4a,b and Supplementary Figs 6d,e and 7a,b ). Addition of Erlotinib inhibits transcriptional activation of IRF3 demonstrating that it is driven by EGFR. Addition of EGF also results in a loss of IRF3 transcriptional activity consistent with our results investigating the expression of IRF3 target genes. Furthermore, Cetuximab failed to inhibit constitutive EGFR-mediated activation of IRF3 in reporter assays in U251EGFR and MDAMB468 cells, further supporting a property of constitutive EGFR signalling ( Fig. 4c and Supplementary Fig. 8a ). Also, a kinase-inactive EGFR mutant failed to activate IRF3 transcriptional activity arguing against a nonspecific effect of EGFR overexpression ( Fig. 4d ). 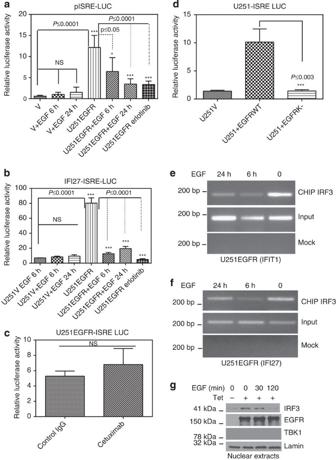Figure 4: Constitutive EGFR signalling activates IRF3 transcriptional activity. (a) The transcriptional activity of IRF3 was examined by using a synthetic pISRE-Luc reporter in U251EGFR cells using a dual luciferase assay. The activity of IRF3 is high in U251EGFR cells compared with U251V (vector-transfected cells). Addition of EGF leads to a statistically significant decrease in reporter activity. Furthermore, Erlotinib also downregulates reporter activity, indicating that the high IRF3 transcriptional activity in the absence of EGF is driven by EGFR. (b) The same experiment asawas conducted in U251EGFR cell using an IFI27-Luc reporter. (c) The EGFR-induced transcriptional activity of IRF3 is not blocked by Cetuximab compared with control IgG in U251EGFR cells. (d) A kinase-inactive EGFR (EGFRK-) fails to activate the pISRE-Luc reporter in U251 cells, whereas the EGFRwt efficiently activates the reporter. Data fora–dwere analysed by one-way ANOVA followed by Tukey’s multiple comparison test. (e) A ChIP assay examining IFIT1 promoter occupancy by IRF3 in U251EGFR cells with or without EGF. IRF3 promoter binding can be detected in the absence of EGF and decreases by 6 h of EGF stimulation and remains decreased 24 h after EGF treatment. (f) A ChIP assay examining IFI27 promoter occupancy by IRF3 in U251EGFR cells with or without EGF. IRF3 promoter binding can be detected in the absence of EGF and decreases by 6 h of EGF stimulation. Cells were serum starved and cultured in serum-free DMEM overnight for all experiments. The EGF concentration used was 50 ng ml−1. (g) We examined the nuclear localization of EGFR, IRF3 and TBK1 in U251 cells conditionally expressing EGFR in response to tetracycline. Cells were treated with tetracycline for 24 h and then exposed to EGF (50 ng ml−1) for the time points indicated. Error bars represent the means±standard deviations of three independent experiments. Data were analysed by one-way ANOVA followed by Tukey’s multiple comparison test. *P≤0.05, **P≤0.01, ***P≤0.001. Figure 4: Constitutive EGFR signalling activates IRF3 transcriptional activity. ( a ) The transcriptional activity of IRF3 was examined by using a synthetic pISRE-Luc reporter in U251EGFR cells using a dual luciferase assay. The activity of IRF3 is high in U251EGFR cells compared with U251V (vector-transfected cells). Addition of EGF leads to a statistically significant decrease in reporter activity. Furthermore, Erlotinib also downregulates reporter activity, indicating that the high IRF3 transcriptional activity in the absence of EGF is driven by EGFR. ( b ) The same experiment as a was conducted in U251EGFR cell using an IFI27-Luc reporter. ( c ) The EGFR-induced transcriptional activity of IRF3 is not blocked by Cetuximab compared with control IgG in U251EGFR cells. ( d ) A kinase-inactive EGFR (EGFRK-) fails to activate the pISRE-Luc reporter in U251 cells, whereas the EGFRwt efficiently activates the reporter. Data for a – d were analysed by one-way ANOVA followed by Tukey’s multiple comparison test. ( e ) A ChIP assay examining IFIT1 promoter occupancy by IRF3 in U251EGFR cells with or without EGF. IRF3 promoter binding can be detected in the absence of EGF and decreases by 6 h of EGF stimulation and remains decreased 24 h after EGF treatment. ( f ) A ChIP assay examining IFI27 promoter occupancy by IRF3 in U251EGFR cells with or without EGF. IRF3 promoter binding can be detected in the absence of EGF and decreases by 6 h of EGF stimulation. Cells were serum starved and cultured in serum-free DMEM overnight for all experiments. The EGF concentration used was 50 ng ml −1 . ( g ) We examined the nuclear localization of EGFR, IRF3 and TBK1 in U251 cells conditionally expressing EGFR in response to tetracycline. Cells were treated with tetracycline for 24 h and then exposed to EGF (50 ng ml −1 ) for the time points indicated. Error bars represent the means±standard deviations of three independent experiments. Data were analysed by one-way ANOVA followed by Tukey’s multiple comparison test. * P ≤0.05, ** P ≤0.01, *** P ≤0.001. Full size image Next, we performed chromatin immunoprecipitation (ChIP) experiments to investigate binding of IRF3 to its target gene promoters. We examined binding of IRF3 to the promoters of IFI27 and IFIT1 in U251EGFR, U87EGFR and MDAMB468 cells in the presence or absence of EGF. We find that IRF3 occupies the IFIT1 and IFI27 promoters in the absence of EGF in all three cell lines. Addition of EGF decreased the binding of IRF3 to the promoter regions of both IFIT1 and IFI27 in U251EGFR cells ( Fig. 4e,f ). A similar result was obtained in MDAMB468 and U87EGFR cells ( Supplementary Fig. 8b–e ). These experiments support a model in which EGFR activates IRF3 in the absence of ligand and this activation is lost with addition of EGF. Next, we examined the localization of IRF3, TBK1 and EGFR in U251 cells conditionally expressing EGFR in response to tetracycline. Increased EGFR expression without ligand exposure leads to increased nuclear localization of EGFR and IRF3, whereas TBK1 is not detected in the nucleus. When EGF is added, nuclear localization of IRF3 decreases over time, whereas there is no change in the amount of nuclear EGFR ( Fig. 4g ). EGFR-mediated IRF3 activation is not mediated by ER stress IRF3 can be activated by endoplasmic reticulum (ER) stress [30] . We examined the possibility that the activation of IRF3 in EGFR-overexpressing cells may result from ER stress and the unfolded protein response secondary to EGFR protein overexpression rather than specific EGFR signalling. Overexpression of another cysteine-rich membrane protein, the LDL receptor, in U251MG cells failed to upregulate IFIT1 and IFI27 ( Supplementary Fig. 8f–h ). Next, we examined whether EGFR overexpression results in increased ER stress and whether the presence of EGF affects it. We examined the phosphorylation of EIF2α as a readout for PERK activation. EGFR overexpression in the absence of ligand does not result in increased EIF2α activation in either U251EGFR or U87EGFR cells compared with vector-transfected cells. Adding EGF results in a small increase in phosphorylation of EIF2α in U251EGFR and U87EGFR cells ( Fig. 5a and Supplementary Fig. 9a ). Similarly, splicing of XBP-1, another measure of ER stress, is not detectable in EGFR-overexpressing cells by western blot or reverse transcription–PCR unless EGF is added to cells ( Fig. 5a and Supplementary Fig. 9b,c ), whereas the expression of BiP/GRP78, a protein known to be upregulated by ER stress, is unchanged ( Fig. 5a and Supplementary Fig. 9b ). These data argue against an increase in ER stress upon EGFR overexpression in the absence of ligand, suggesting that constitutive EGFR signalling-induced IRF3 activation and gene induction are independent of ER stress. Erlotinib has no effect on markers of ER stress ( Fig. 5a and Supplementary Fig. 9a,b ). Next, we examined whether inhibition of the three major arms of the unfolded protein response (UPR) would inhibit constitutive EGFR signalling-induced IRF3 activation. First, PRKR-like endoplasmic reticulum kinase (PERK) inhibition using GSK 2606414 failed to inhibit EGFR-induced IRF3 activation and IFIT1 and IFI27 induction, whereas the PERK inhibitor efficiently inhibited thapsigargin-induced EIF2α phosphorylation ( Fig. 5b,c and Supplementary Figs 9d–g,10a ). Next, ATF6 inhibition using 4-(2-aminoethyl) benzenesulfonyl fluoride (AEBSF) also failed to inhibit EGFR-induced IRF3 activation and IFIT1 and IFI27 induction ( Fig. 5d and Supplementary Figs 9h,10b–e ), whereas AEBSF efficiently blocked thapsigargin-induced activation of a ATF6 promoter, p5xATF6GL3 ( Fig. 5e ). Finally, siRNA knockdown of XBP-1 failed to prevent EGFR-induced IRF3 activation and gene induction ( Fig. 5f–h and Supplementary Fig. 10f–h ). Thus, we conclude that constitutive EGFR signalling is independent of ER stress. 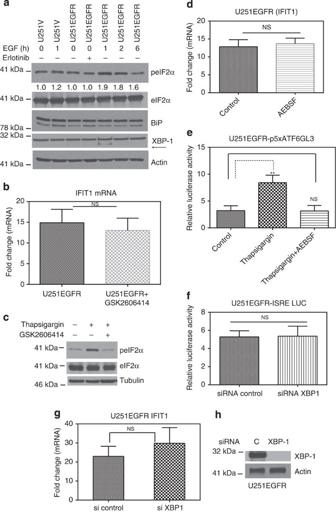Figure 5: EGFR constitutive signalling is independent of ER stress. (a) U251V cells (transfected with empty vector) and U251EGFR cells were examined for phosphorylation of EIF2α. EGF or Erlotinib was added as indicated followed by lysate preparation and western blot with phospo-EIF2α antibodies. Densitometry was performed to quantify the pEIF2α signal. Splicing of XBP-1 or level of BiP were examined by western blot in U251EGFR cells. Splicing of XBP-1 can only be detected in EGF-treated cells. BiP levels are unchanged. (b) U251EGFR cells were treated with a PERK inhibitor, GSK 2606414 (1 μM) overnight followed by RNA extraction and quantitative PCR (qPCR) for IFIT1. GSK 2606414 fails to prevent EGFR-mediated IFIT1 induction. (c) GSK 2606414 efficiently inhibits thapsigargin (0.5 μM for 6 h)-induced phosphorylation of EIF2α as shown in the western blot with phospo-EIF2α antibodies. (d) U251EGFR cells were treated with an ATF6 inhibitor, AEBSF (300 μM) overnight followed by RNA extraction and qPCR for IFIT1. AEBSF fails to prevent EGFR-mediated IFIT1 induction. (e) AEBSF (300 μM) efficiently inhibits thapsigargin-induced ATF6 promoter activity in a reporter assay. (f) Silencing XBP-1 fails to prevent EGFR-induced activation of IRF3-mediated transcriptional activity assessed using a synthetic pISRE-Luc reporter. (g) Silencing XBP-1 fails to prevent EGFR-induced induction of IFIT1 in U251EGFR cells. (h) Effective silencing of XBP-1 is demonstrated in U251EGFR cells by western blot. Error bars represent the means±standard deviations of three independent experiments. Data were analysed by one-way ANOVA followed by Tukey’s multiple comparison test. *P≤0.05, **P≤0.01, ***P≤0.001. Figure 5: EGFR constitutive signalling is independent of ER stress. ( a ) U251V cells (transfected with empty vector) and U251EGFR cells were examined for phosphorylation of EIF2α. EGF or Erlotinib was added as indicated followed by lysate preparation and western blot with phospo-EIF2α antibodies. Densitometry was performed to quantify the pEIF2α signal. Splicing of XBP-1 or level of BiP were examined by western blot in U251EGFR cells. Splicing of XBP-1 can only be detected in EGF-treated cells. BiP levels are unchanged. ( b ) U251EGFR cells were treated with a PERK inhibitor, GSK 2606414 (1 μM) overnight followed by RNA extraction and quantitative PCR (qPCR) for IFIT1. GSK 2606414 fails to prevent EGFR-mediated IFIT1 induction. ( c ) GSK 2606414 efficiently inhibits thapsigargin (0.5 μM for 6 h)-induced phosphorylation of EIF2α as shown in the western blot with phospo-EIF2α antibodies. ( d ) U251EGFR cells were treated with an ATF6 inhibitor, AEBSF (300 μM) overnight followed by RNA extraction and qPCR for IFIT1. AEBSF fails to prevent EGFR-mediated IFIT1 induction. ( e ) AEBSF (300 μM) efficiently inhibits thapsigargin-induced ATF6 promoter activity in a reporter assay. ( f ) Silencing XBP-1 fails to prevent EGFR-induced activation of IRF3-mediated transcriptional activity assessed using a synthetic pISRE-Luc reporter. ( g ) Silencing XBP-1 fails to prevent EGFR-induced induction of IFIT1 in U251EGFR cells. ( h ) Effective silencing of XBP-1 is demonstrated in U251EGFR cells by western blot. Error bars represent the means±standard deviations of three independent experiments. Data were analysed by one-way ANOVA followed by Tukey’s multiple comparison test. * P ≤0.05, ** P ≤0.01, *** P ≤0.001. Full size image Constitutive EGFR-induced phosphorylation of IRF3 and TBK1 The transcriptional activity of IRF3 is regulated by phosphorylation of serine residues in the C-terminal regulatory domain. The Tank-binding kinase (TBK1) and IKKε have been identified as the kinases that phosphorylate IRF3 (ref. 24 ). TBK1 is also regulated by phosphorylation of serine 172 by autophosphorylation or by IKKβ [31] . We examined whether constitutive or ligand-induced EGFR signalling induces phosphorylation of IRF3 and/or TBK1. Indeed, we find constitutive serine phosphorylation of IRF3 in U251EGFR cells that is abolished by Erlotinib and by EGF, indicating that it is EGFR driven and also a feature of constitutive EGFR signalling ( Fig. 6a ). 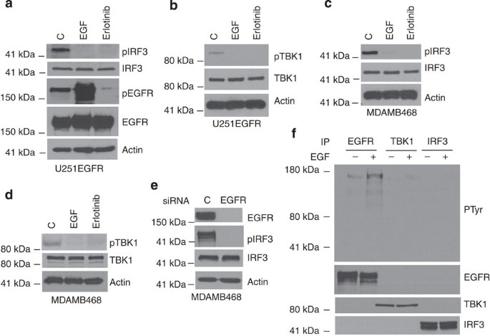Figure 6: Constitutive EGFR signalling results in IRF3 and TBK1 phosphorylation. (a) IRF3 is phosphorylated in U251EGFR cells in the absence of ligand. When EGF is added (50 ng ml−1for 15 min), there is a rapid decrease in IRF3 phosphorylation. Erlotinib also inhibits IRF3 phosphorylation. (b) TBK1 is phosphorylated in U251EGFR cells in the absence of ligand. When EGF is added, there is a rapid decrease in TBK1 phosphorylation. (c) Similarly, IRF3 is phosphorylated in MDAMB468 cells and exposure to EGF or Erlotinib downregulates IRF3 phosphorylation. (d) TBK1 is phosphorylated in MDAMB468 cells and exposure to EGF or Erlotinib downregulates TBK1 phosphorylation. (e) siRNA knockdown of EGFR in MDAMB468 cells results in a loss of IRF3 phosphorylation compared with control siRNA (C). (f) Neither IRF3 nor TBK1 are tyrosine phosphorylated in EGFR-overexpressing cells. We immunoprecipitated IRF3 or TBK1 in U251EGFR cells followed by western blot with phosphotyrosine antibodies. As a positive control, we immunoprecipitated EGFR. Cells were serum starved and cultured in serum-free DMEM overnight for all experiments. The EGF concentration used was 50 ng ml−1. Figure 6a also shows a low level of EGFR tyrosine phosphorylation in the absence of ligand. In addition to IRF3, TBK1 is also phosphorylated in U251EGFR cells. Addition of EGF or Erlotinib abolishes TBK1 serine 172 phosphorylation in U251EGFR cells ( Fig. 6b ). Similarly, IRF3 and TBK1 are phosphorylated in MDAMD468 cells and exposure to EGF or Erlotinib abolishes this phosphorylation ( Fig. 6c,d ). Also, silencing EGFR in MDAMB468 cells results in a loss of IRF3 activation ( Fig. 6e ). We did not detect tyrosine phosphorylation of IRF3 or TBK1 in response to EGFR overexpression with or without EGF. The experiment was conducted by immunoprecipitating TBK1 and IRF3 (or EGFR as a positive control) from denatured EGFR-overexpressing cell lysates followed by immunoblotting with a phosphotyrosine antibody ( Fig. 6f ). Figure 6: Constitutive EGFR signalling results in IRF3 and TBK1 phosphorylation. ( a ) IRF3 is phosphorylated in U251EGFR cells in the absence of ligand. When EGF is added (50 ng ml −1 for 15 min), there is a rapid decrease in IRF3 phosphorylation. Erlotinib also inhibits IRF3 phosphorylation. ( b ) TBK1 is phosphorylated in U251EGFR cells in the absence of ligand. When EGF is added, there is a rapid decrease in TBK1 phosphorylation. ( c ) Similarly, IRF3 is phosphorylated in MDAMB468 cells and exposure to EGF or Erlotinib downregulates IRF3 phosphorylation. ( d ) TBK1 is phosphorylated in MDAMB468 cells and exposure to EGF or Erlotinib downregulates TBK1 phosphorylation. ( e ) siRNA knockdown of EGFR in MDAMB468 cells results in a loss of IRF3 phosphorylation compared with control siRNA (C). ( f ) Neither IRF3 nor TBK1 are tyrosine phosphorylated in EGFR-overexpressing cells. We immunoprecipitated IRF3 or TBK1 in U251EGFR cells followed by western blot with phosphotyrosine antibodies. As a positive control, we immunoprecipitated EGFR. Cells were serum starved and cultured in serum-free DMEM overnight for all experiments. The EGF concentration used was 50 ng ml −1 . Full size image EGFR-associated protein complexes To investigate the mechanism of how EGFR activates IRF3, we examined whether the EGFR associates with IRF3 in U251EGFR cells. We find that IRF3 forms a complex with the EGFR. Importantly, the EGFR–IRF3 complex is disrupted when EGF is added ( Fig. 7a ). EGFR also forms a complex with TBK1 that is disrupted by EGF ( Fig. 7b ). Importantly, IRF3 also forms a complex with TBK1 that is dependent on constitutive EGFR activity. There is a loss of the IRF3–TBK1 association when EGFR kinase activity is inhibited with Erlotinib. In addition, exposure of cells to EGF also results in a loss of IRF3–TBK1 association ( Fig. 7c ). Similar results were detected in MDABM468 ( Fig. 7d–f ) and U87EGFR cells ( Supplementary Fig. 11a–c ). Thus, these data suggest that EGFR recruits TBK1 to IRF3 and both IRF3 and TBK1 to the EGFR forming a ternary complex at the EGFR. We estimate that about 10% of the cellular IRF3 is complexed to the EGFR, and about 5% of the phosphorylated IRF3 is complexed to the EGFR as shown in Fig. 7h–i . 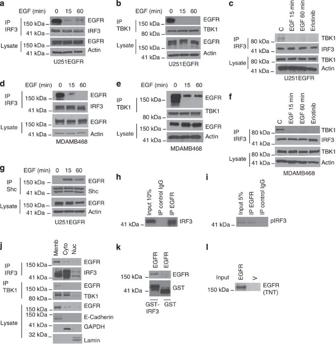Figure 7: EGFR forms a signalling complex with IRF3 and TBK1. (a) EGFR co-immunoprecipitates with IRF3 in U251EGFR cells in the absence of EGF. When EGF is added there is a rapid loss of the EGFR–IRF3 association. (b) Similarly, the EGFR co-immunoprecipitates with TBK1 in U251EGFR cells. When EGF is added, there is a rapid loss of the EGFR–TBK1 association. (c) TBK1 is associated with IRF3 in U251EGFR cells in the absence of EGF. When EGF is added to cells, there is a rapid decrease in TBK–IRF3 association. The TBK1–IRF3 association is also disrupted when Erlotinib is used suggesting that it is EGFR driven. C refers to control vehicle (PBS). (d) EGFR co-immunoprecipitates with IRF3 in MDAMB468 cells in the absence of EGF. When EGF is added there is a rapid loss of the EGFR-IRF3 association. (e) Similarly, the EGFR co-immunoprecipitates with TBK1 in MDAMB468 cells. When EGF is added there is a rapid loss of the EGFR–TBK1 association. (f) TBK1 is associated with IRF3 in MDAMB468 cells in the absence of EGF. When EGF is added to cells, there is a rapid decrease in TBK–IRF3 association. The TBK1–IRF3 association is also disrupted when Erlotinib is used suggesting that it is EGFR driven. (g) In contradistinction to IRF3 and TBK1, Shc becomes associated with the EGFR only when EGF is added to U251EGFR cells. (h) About 10% of IRF3 is associated with the EGFR. (i) About 5% of phospho-IRF3 is associated with the EGFR. (j) EGFR associates with IRF3 and TBK1 in the membrane fraction. Membrane, cytosolic or nuclear fractions were prepared from U251EGFR cells. Immunoprecipitation was conducted with IRF3 or TBK1 antibody followed by western blot with EGFR. E-Cadherin, glyceraldehyde 3-phosphate dehydrogenase (GAPDH) and lamin blots were done to test purity of various fractions. Cells were serum starved and cultured in serum-free DMEM overnight for all experiments. The EGF concentration used was 50 ng ml−1. (k)In vitrotranscribed and translated EGFR was incubated with GST-IRF3 or GST alone followed by western blot with EGFR. (l)In vitrotranscribed and translated EGFR. V, empty vector. Figure 7: EGFR forms a signalling complex with IRF3 and TBK1. ( a ) EGFR co-immunoprecipitates with IRF3 in U251EGFR cells in the absence of EGF. When EGF is added there is a rapid loss of the EGFR–IRF3 association. ( b ) Similarly, the EGFR co-immunoprecipitates with TBK1 in U251EGFR cells. When EGF is added, there is a rapid loss of the EGFR–TBK1 association. ( c ) TBK1 is associated with IRF3 in U251EGFR cells in the absence of EGF. When EGF is added to cells, there is a rapid decrease in TBK–IRF3 association. The TBK1–IRF3 association is also disrupted when Erlotinib is used suggesting that it is EGFR driven. C refers to control vehicle (PBS). ( d ) EGFR co-immunoprecipitates with IRF3 in MDAMB468 cells in the absence of EGF. When EGF is added there is a rapid loss of the EGFR-IRF3 association. ( e ) Similarly, the EGFR co-immunoprecipitates with TBK1 in MDAMB468 cells. When EGF is added there is a rapid loss of the EGFR–TBK1 association. ( f ) TBK1 is associated with IRF3 in MDAMB468 cells in the absence of EGF. When EGF is added to cells, there is a rapid decrease in TBK–IRF3 association. The TBK1–IRF3 association is also disrupted when Erlotinib is used suggesting that it is EGFR driven. ( g ) In contradistinction to IRF3 and TBK1, Shc becomes associated with the EGFR only when EGF is added to U251EGFR cells. ( h ) About 10% of IRF3 is associated with the EGFR. ( i ) About 5% of phospho-IRF3 is associated with the EGFR. ( j ) EGFR associates with IRF3 and TBK1 in the membrane fraction. Membrane, cytosolic or nuclear fractions were prepared from U251EGFR cells. Immunoprecipitation was conducted with IRF3 or TBK1 antibody followed by western blot with EGFR. E-Cadherin, glyceraldehyde 3-phosphate dehydrogenase (GAPDH) and lamin blots were done to test purity of various fractions. Cells were serum starved and cultured in serum-free DMEM overnight for all experiments. The EGF concentration used was 50 ng ml −1 . ( k ) In vitro transcribed and translated EGFR was incubated with GST-IRF3 or GST alone followed by western blot with EGFR. ( l ) In vitro transcribed and translated EGFR. V, empty vector. Full size image To identify the cellular compartment in which the EGFR and IRF3 interact in U251EGFR cells, we undertook cellular fractionation studies and examined co-immunoprecipitation of EGFR and IRF3 in membrane, cytoplasmic and nuclear lysates. We find that EGFR and IRF3 associate primarily in the plasma membrane as shown in Fig. 7j . However, in U251V cells, almost all of the IRF3 is cytoplasmic ( Supplementary Fig. 11e ), suggesting that IRF3 is recruited to the membrane compartment by the EGFR in U251EGFR cells. Also, EGFR may directly associate with IRF3 as shown in Fig. 7k,l . In this experiment, glutathione S-transferase (GST)-IRF3 was incubated with in vitro transcribed and translated EGFR. EGFR associates with GST-IRF3 but not with GST alone in vitro . We cannot detect IKKε expression in U251EGFR and U87EGFR cells by western blot ( Supplementary Fig. 11f ), suggesting that IKKε does not play a role in EGFR-mediated IRF3 activation. This EGFR signalling platform described above is formed in the absence of ligand. Importantly, addition of EGF results in a rapid dissociation of this signalling platform. The ligand-activated EGFR is known to bind a number of secondary signalling proteins. These include the adaptor protein Shc, which has a role coupling growth factor signalling to mitogen-activated protein kinase activation [32] . Although IRF3 and TBK1 dissociate from the EGFR upon ligand binding, Shc becomes associated with the EGFR only when EGF is added ( Fig. 7f and Supplementary Fig. 11d ). The switch of EGFR-associated proteins with ligand may underlie the distinct and mutually exclusive nature of constitutive and ligand-induced signalling. Constitutive EGFR activates the interferon pathway IFIT1 and IFI27 are interferon-inducible genes and EGFR-mediated activation of IRF3 could lead to induction of IFN-β followed by activation of the type I interferon receptor culminating in transcription of IFN-α and interferon-inducible genes. We examined first if the levels of IFN-β and IFN-α were upregulated in EGFR-overexpressing cells. Consistent with our data showing EGFR activates IRF3 in the absence of ligand, we find high levels of IFN-β and IFN-α mRNA in EGFR-overexpressing cells. When EGF or erlotinib is added there is a decrease in IFN-β and IFN-α mRNA levels as shown in Fig. 8a,b and Supplementary Fig. 12a,b . Increased levels of IFN-β can also be detected in supernatants from EGFR-overexpressing cells ( Fig. 8c and Supplementary Fig. 12c ). IRF7 is another IFN-inducible gene that plays an important role in IFN signalling. However, we could not detect expression of IRF7 in U251EGFR and U87EGFR cells ( Supplementary Fig. 12d ). The secretion of IFN-β results in activation of the JAK-STAT1/2 pathway and we examined whether EGFR overexpression results in phosporylation of STAT1. As shown in Fig. 8d , STAT1 is activated in EGFR-overexpressing cells and addition of EGF to these cells results in attenuation of STAT1 phosphorylation. Next, we examined the effect of specific JAK tyrosine kinase inhibitors on EGFR-mediated induction of IFIT1 and IFI27. We have found that Ruxolitinib suppresses IFI27 and IFIT1 mRNA expression in EGFR-overexpressing cells as does as Tofacitinib ( Fig. 8e–g and Supplementary Fig. 12E–G and 13a–c ). However, the JAK inhibitors have no effect on EGF-mediated ERK or Akt activation ( Supplementary Fig. 13d,e ). A previous study has reported an interaction between TLR3 and the EGFR [33] . However, TLR3 is not expressed in U251EGFR or U87EGFR cells ( Supplementary Fig. 14a ) arguing against a role for TLR3 in constitutive EGFR signalling. 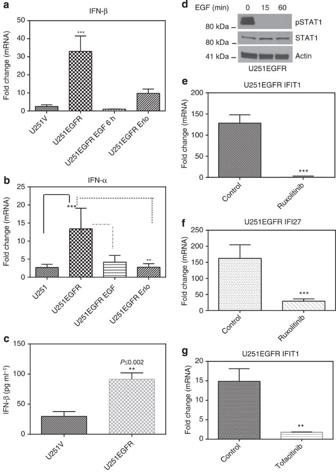Figure 8: Constitutive EGFR signalling activates the interferon pathway. (a) EGFR overexpression leads to increased mRNA for IFN-β compared with vector-transfected cells. Addition of EGF or Erlotinib leads to a loss of this increase in IFN-β in EGFR-overexpressing cells. (b) EGFR overexpression leads to increased mRNA for IFN-α compared with vector-transfected cells. Addition of EGF or Erlotinib leads to decreased IFN-α in EGFR-overexpressing cells. (c) An ELISA done on supernatants from U251EGFR or vector-transfected cells shows that EGFR overexpression leads to increased IFN-β at a protein level. (d) STAT1 is phosphorylated in U251EGFR cells. This phosphorylation is lost when EGF (15 min) is added to cells. (e,f) U251EGFR cells were incubated with Ruxolinitib (1 μM) overnight followed by extraction of RNA and quantitative PCR (qPCR) for IFIT1 or IFI27. (g) U251EGFR cells were incubated with Tofacitinib (300 nM) overnight followed by extraction of RNA and qPCR. Cells were serum starved and cultured in serum-free DMEM overnight for all experiments. The EGF concentration used was 50 ng ml−1. Error bars represent the means±standard deviations of three independent experiments. Data were analysed by one-way ANOVA followed by Tukey’s multiple comparison test. *P≤0.05,**P≤0.01, ***P≤0.001. Figure 8: Constitutive EGFR signalling activates the interferon pathway. ( a ) EGFR overexpression leads to increased mRNA for IFN-β compared with vector-transfected cells. Addition of EGF or Erlotinib leads to a loss of this increase in IFN-β in EGFR-overexpressing cells. ( b ) EGFR overexpression leads to increased mRNA for IFN-α compared with vector-transfected cells. Addition of EGF or Erlotinib leads to decreased IFN-α in EGFR-overexpressing cells. ( c ) An ELISA done on supernatants from U251EGFR or vector-transfected cells shows that EGFR overexpression leads to increased IFN-β at a protein level. ( d ) STAT1 is phosphorylated in U251EGFR cells. This phosphorylation is lost when EGF (15 min) is added to cells. ( e , f ) U251EGFR cells were incubated with Ruxolinitib (1 μM) overnight followed by extraction of RNA and quantitative PCR (qPCR) for IFIT1 or IFI27. ( g ) U251EGFR cells were incubated with Tofacitinib (300 nM) overnight followed by extraction of RNA and qPCR. Cells were serum starved and cultured in serum-free DMEM overnight for all experiments. The EGF concentration used was 50 ng ml −1 . Error bars represent the means±standard deviations of three independent experiments. Data were analysed by one-way ANOVA followed by Tukey’s multiple comparison test. * P ≤0.05,** P ≤0.01, *** P ≤0.001. Full size image EGFR signalling influences sensitivity to virus infection As noted, constitutive EGFR signalling activates IRF3 and induces IRF3-dependent transcription of downstream genes. To examine possible biological outcomes of EGFR-mediated IRF3 activation, we infected adenovirus-GFP into U251EGFR and U87EGFR cells in the presence or absence of EGF. Previous studies have shown that adenovirus infection activates an inflammatory response and activates IRF3 (refs 34 , 35 ). Surprisingly, we find that EGF-treated cells undergo a significant amount of cell death when exposed to adenovirus-GFP ( Fig. 9a ) compared with cells not treated with EGF. We also undertook an Annexin-propidium iodide fluorescence-activated cell sorting (FACS) experiment in these cells and confirmed that EGF treatment results in an increased sensitivity to adenovirus ( Fig. 9b,c ). Thus, infection with adenovirus results in cell death in the presence of EGF, consistent with the loss of IRF3 transcriptional activity. The cell death has features of both apoptosis and necrosis. We also determined the effect of Erlotinib or Cetuximab in U251EGFR cells. We find that Erlotinib or Cetuximab results in a loss of the EGF-mediated sensitivity to adenovirus ( Fig. 9b ). We also compared the sensitivity of U251EGFR to U251V cells and U87EGFR to U87V cells to determine if EGFR overexpression alters sensitivity to virus infection. We find that EGFR overexpression confers resistance to adenovirus toxicity ( Supplementary Fig. 15a,b ). However, adding EGF turns off IRF3 transcriptional activity and antiviral immunity in these cells resulting in an unexpected vulnerability to adenovirus-induced cell death in these cells. 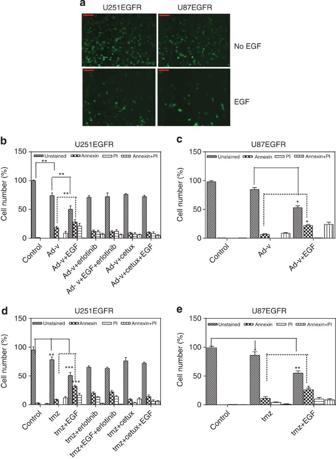Figure 9: Ligand-activated EGFR increases sensitivity to virus- and chemotherapy-mediated cell death. (a) U251 and U87EGFR cells were infected with adenovirus-GFP at an MOI of 10. Cells were examined with immunofluorescence microscopy after 24 h. EGF (50 ng ml−1) or control vehicle were added at the time of adenovirus infection. (b,c) U251EGFR or U87EGFR cells were infected with adenovirus following by an Annexin-FACS assay for detecting cell death. EGF (50 ng ml−1) was added at the time of infection for 24 h and leads to a statistically significant increase in Annexin and PI positive cells compared to cells exposed to adenovirus alone. (d) U251EGFR cells were exposed to EGF or control vehicle and temozolomide (50 μM) for 24 h and an Annexin-FACS assay was performed. In ‘Control’ cells are treated with control vehicle (PBS). Temozolomide alone induces cell death in these cells. The cell death is strikingly amplified when cells are pretreated with EGF (P≤0.001). (e) A similar experiment was conducted in U87EGFR cells with a similar result (P≤0.001). Data were analysed by one-way ANOVA followed by Tukey’s Multiple Comparison test. Cells were serum starved and cultured in serum-free DMEM overnight for all experiments. The EGF concentration used was 50 ng ml−1. Error bars represent the means±standard deviations of three independent experiments. Data were analysed by one-way ANOVA followed by Tukey’s multiple comparison test. *P≤0.05,**P≤0.01, ***P≤0.001. Figure 9: Ligand-activated EGFR increases sensitivity to virus- and chemotherapy-mediated cell death. ( a ) U251 and U87EGFR cells were infected with adenovirus-GFP at an MOI of 10. Cells were examined with immunofluorescence microscopy after 24 h. EGF (50 ng ml −1 ) or control vehicle were added at the time of adenovirus infection. ( b , c ) U251EGFR or U87EGFR cells were infected with adenovirus following by an Annexin-FACS assay for detecting cell death. EGF (50 ng ml −1 ) was added at the time of infection for 24 h and leads to a statistically significant increase in Annexin and PI positive cells compared to cells exposed to adenovirus alone. ( d ) U251EGFR cells were exposed to EGF or control vehicle and temozolomide (50 μM) for 24 h and an Annexin-FACS assay was performed. In ‘Control’ cells are treated with control vehicle (PBS). Temozolomide alone induces cell death in these cells. The cell death is strikingly amplified when cells are pretreated with EGF ( P ≤0.001). ( e ) A similar experiment was conducted in U87EGFR cells with a similar result ( P ≤0.001). Data were analysed by one-way ANOVA followed by Tukey’s Multiple Comparison test. Cells were serum starved and cultured in serum-free DMEM overnight for all experiments. The EGF concentration used was 50 ng ml −1 . Error bars represent the means±standard deviations of three independent experiments. Data were analysed by one-way ANOVA followed by Tukey’s multiple comparison test. * P ≤0.05,** P ≤0.01, *** P ≤0.001. Full size image EGFR signalling influences sensitivity to chemotherapy Previous studies have reported that aberrant EGFR signalling reduces sensitivity to radiation and chemotherapy. This is not surprising considering that EGFR activates a number of survival signals. We compared the sensitivity of EGFR-expressing cells in the absence or presence of EGF to temozolomide, a first-line chemotherapy drug used in the treatment of patients with GBM. Surprisingly, we find that ligand-activated U251EGFR and U87EGFR cells are more vulnerable to the effect of temozolomide compared with cells not exposed to ligand. In this experiment, cells were exposed to EGF for 24 h followed by temozolomide for 48 h. The exposure to EGF sensitizes these cells to temozolomide in a manner analogous to what has been described for the Met receptor [36] . We conducted an Annexin-propidium iodide FACS assay to examine cell death following treatment with temozolomide. In both U251EGFR and U87EGFR cell lines, temozolomide induces more cell death when cells are exposed to EGF ( Fig. 9d,e ). We also determined the effect of Erlotinib or Cetuximab in U251EGFR cells. We find that Erlotinib or Cetuximab results in a decrease of the EGF-mediated sensitivity to temozolomide ( Fig. 9d ). We also compared the sensitivity of U251EGFR to U251V cells and U87EGFR to U87V cells to determine whether EGFR overexpression alters sensitivity to temozolomide. We find that EGFR overexpression confers resistance to the induction of cell death by temozolomide ( Supplementary Fig. 16a–c ) in multiple cell lines. Constitutive EGFR signalling in GBM The EGFR is commonly overexpressed in GBM and we examined whether evidence of constitutive EGFR signalling is detectable in GBM. We hypothesized that in EGFR-expressing tumours, when ligand is low, we would detect evidence of constitutive EGFR signalling as determined by elevated expression of the downstream genes IFIT1 and IFI27 . Conversely, in tumours in which the ligand expression is high, we would expect expression of IFIT1 and IFI27 to be low. To test this hypothesis, we examined 27 GBM tumours for EGFR, the EGFR ligand TGF-α, and IFIT1 and IFI27 levels by quantitative real-time PCR ( Fig. 10 ). TGF-α was chosen because a number of studies have shown it to be the major EGFR ligand expressed in GBM [27] , [28] , [37] . Among EGFR-overexpressing tumours ( Fig. 10a,b and Supplementary Fig. 17d ) that have low TGF-α levels, we find that all 13 GMBs have a high level of IFIT1 and IFI27, consistent with constitutive EGFR signalling in GBMs ( Fig. 10c,d ). Among the nine EGFR-overexpressed tumours that have high TGF-α levels, IFIT1 and IFI27 levels are generally low ( Fig. 10e,f ). The negative correlation between TGF-α and IFI27 and IFIT1 in EGFR-overexpressing tumours is statistically highly significant (Spearman nonparametric correlation for TGF-α and IFI27: P <0.0001, r =−0.75; for TGF-α and IFIT1: P <0.0001, r =−0.74). Among the five GBMs with low EGFR expression, IFIT1 and IFI27 levels are low, whereas TGF-α levels are mixed ( Supplementary Fig. 17c ). These data provide strong evidence of constitutive EGFR signalling in human GBM. 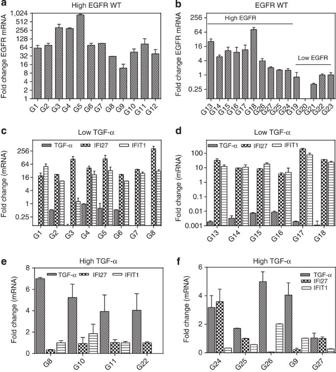Figure 10: Constitutive EGFR signalling in GBM. (a,b) EGFR levels in 27 GBM tumours by real-time quantitative PCR. An arbitrary cutoff of 1 or above was considered to be EGFR overexpression and corresponded well to expression levels of EGFR on western blot (Supplementary Fig. 17D). (c,d) TGF-α, IFIT1 and IFI27 levels in GBMs expressing a low level of TGF-α (less than 1) measured by real-time quantitative PCR. (e,f) TGF-α, IFIT1 and IFI27 levels in GBM tumours expressing a high level of TGF-α measured by real-time quantitative PCR. Figure 10: Constitutive EGFR signalling in GBM. ( a , b ) EGFR levels in 27 GBM tumours by real-time quantitative PCR. An arbitrary cutoff of 1 or above was considered to be EGFR overexpression and corresponded well to expression levels of EGFR on western blot ( Supplementary Fig. 17D ). ( c , d ) TGF-α, IFIT1 and IFI27 levels in GBMs expressing a low level of TGF-α (less than 1) measured by real-time quantitative PCR. ( e , f ) TGF-α, IFIT1 and IFI27 levels in GBM tumours expressing a high level of TGF-α measured by real-time quantitative PCR. Full size image Although various EGFR mutants are known to be constitutively active and their downstream signals are relatively well studied, constitutive activation of the EGFR wild type is not well understood. It is known that EGFR overexpression results in tyrosine phosphorylation and constitutive activation of the EGFR. However, the downstream signals resulting from constitutive activation of the EGFR are unknown. Here we show that constitutive EGFR signalling does trigger downstream signals and describe a form of constitutive or non-canonical EGFR signalling that includes activation of the transcription factor IRF3 and transcription of genes involved in innate immunity. However, the overexpressed EGFR does not activate ERK and Akt unless ligand is added. Addition of EGF results in termination of IRF3 activation and gene transcription and activation of the ligand-activated signalling programme with ERK and Akt activation and induction of early genes, suggesting that the constitutive and ligand-induced signalling programmes are distinct and mutually exclusive. Thus, the EGFR oscillates between alternative programmes of signalling depending on the availability of ligand. This bimodal signalling appears to be a property of EGFR overexpression commonly detected in cancer and is not detected at lower levels of EGFR expression. Multiple lines of evidence suggest that EGFR signalling in our experimental model is constitutive and cannot be explained by autocrine or paracrine loops. Addition of exogenous EGF inhibits EGFR-mediated activation of IRF3 and IRF3-dependent gene transcription including IFIT1 and IFI27. Also, Cetuximab, which inhibits ligand binding to the EGFR, fails to inhibit EGFR-mediated activation of IRF3 and IRF3-dependent gene transcription, whereas a mutant EGFRvIII, which does not bind any ligand, upregulates IFIT1 and IRF3. Furthermore, as the ER stress response is known to activate IRF3, we rigorously excluded the possibility that signalling detected upon EGFR overexpression is secondary to ER stress. Signals generated by constitutive EGFR signalling appear to be distinct and mutually exclusive from ligand-activated signals. Our data indicate that the mechanism of differential signalling depends on recruitment of a distinct set of proteins to the EGFR. Thus, in the absence of ligand, the EGFR forms a signalling platform with IRF3 and TBK1. The formation of a ternary complex between these three proteins is suggested by the fact that increased expression of the EGFR results in increased association of TBK1 with its substrate IRF3 and the fact that both proteins are complexed with the EGFR. This signalling platform is detected in multiple cancer cell lines and localizes to the cell membrane. Addition of EGF results in a rapid dissolution of the EGFR signalling platform and separation of TBK1 and IRF3 from each other and from the EGFR. We propose that formation of the EGFR signalling platform with EGFR, TBK1 and IRF3 results in the phosphorylation and activation of TBK1 and IRF3. The juxtaposition of IRF3 and TBK1 in the EGFR-associated complex presumably facilitates TBK1-mediated phosphorylation of IRF3 leading to its activation. EGFR-mediated activation of IRF3 can also be detected in reporter and ChIP assays and transcription of IRF3-dependent genes. We propose that IRF3 is activated at the cell membrane and then translocates to the nucleus, partly analogous to the model described for EGFR-mediated activation of STAT3 (ref. 38 ). Activation of IRF3 results in transcription of downstream genes involved in antiviral innate immunity, such as IFIT1 and IFI27. Thus, in the absence of ligand, EGFR expression results in significant upregulation of IFIT1 and IFI27. Thus, constitutive or non-canonical EGFR signalling is mediated via an EGFR-IRF3 signalling axis. When cells are exposed to EGF, constitutive EGFR signalling is switched off. This can be detected at several levels. There is a rapid dissociation of the EGFR-TBK-1-IRF3 signalling platform and a loss of TBK1 and IRF3 phosphorylation. In addition, there is a loss of IRF3 transcriptional activity detected in reporter assays and ChIP experiments, and a decrease in the level of EGFR-IRF3-induced genes such as IFIT1 and IFI27. Exposure to EGF results in triggering of a distinct downstream signalling cascade. Ligand-mediated activation of the EGFR is known to recruit a number of downstream signalling proteins that include Shc, Gab1 and Grb2 (ref. 39 ). We looked at the association of one of these proteins (Shc) with the EGFR in U251EGFR and U87EGFR cells. As expected, in the absence of EGF, Shc is not associated with the EGFR. However, when the EGFR is activated with ligand, Shc becomes associated with the EGFR. In addition, we detected increased activation of ERK and Akt when cells are exposed to EGF and upregulation of known immediate early genes EGR1 and EGR2. IFIT1 and IFI27 are interferon-inducible genes and IRF3 appears to exert its effects by stimulating transcription of IFN-β followed by the activation of the JAK-STAT1/2 pathway and subsequent transcription of IFN-inducible genes. The engagement of this pathway in constitutive EGFR signalling is suggested by experiments demonstrating that EGFR upregulates IFN-β and IFN-α and results in activation of STAT1. Furthermore, EGFR-mediated induction of IFIT1 and IFI27 is blocked by the specific JAK inhibitors, Ruxolitinib and Tofacitib. Previous studies have indicated that type I interferons may have a complex effect on tumour growth [40] . Also, a recent study has demonstrated a requirement for EGFR in TLR3 signalling in response to viral infection [33] . However, TLR3 is not expressed in U251EGFR and U87EGFR cells and is not required for EGFR-mediated IRF3 activation. The biological effects of constitutive versus ligand-mediated EGFR activation are not well understood. Importantly, we find that cells with constitutively activated EGFR are relatively resistant to adenovirus-mediated toxicity. Thus, constitutive/non-canonical EGFR-mediated activation of IRF3 may confer an advantage during the clonal evolution of tumours, conferring protection to tumours from pathogens infecting the host. EGFR-mediated activation of IRF3 results in the transcription of a number of genes involved in antiviral immunity and the innate immune response. Addition of EGF results in a loss of IRF3-mediated transcriptional activity and unmasks a surprising vulnerability of these cells to adenovirus infection. It is well established that ligand-mediated EGFR activation triggers known oncogenic signals such as ERK and Akt and promotes the malignant phenotype. As ligand-independent and -dependent EGFR signalling trigger distinct signals and possibly distinct biological outcomes, our study highlights the critical importance of ligand in the microenvironment of the tumour. The presence of ligand may also influence sensitivity to chemotherapy, as our findings indicate that EGF-treated cells are more sensitive to temozolomide. Finally, we present data suggesting that constitutive EGFR signalling is activated in GBM. In high EGFR-expressing tumours, we would predict that in tumours with low levels of ligand, constitutive EGFR signalling would be prevalent leading to increased expression of IRF3-mediated gene expression. Indeed, we find that there is an inverse correlation between TGF-α levels and IFIT1 and IFI27 levels in GBMs that express a high level of EGFR. Thus, the presence or absence of ligand in individual tumours may determine signalling networks activated by the EGFR, and, in turn, may have important implications for targeted treatment. Plasmid transfection and generation of cell lines U251MG cells were obtained from Dr Robert Bachoo. U87MG and MDAMB468 cells were obtained from American Type Culture Collection. 429NS cells were provided by Dr Santosh Kesari. The GBM cell lines U251MG was used to generate cell lines conditionally expressing EGFRwt or EGFRvIII using the T-Rex Tet-on system from Invitrogen as we have described previously [26] . U251MG and U87MG cells were transfected with EGFRwt in PcDNA 3.1 and selected in G418 to generate stable cell lines constitutively and stably expressing EGFR. Lipofectamine 2000 (Invitrogen) was used for all transfections. Primary GBM cultures were generated directly from human GBM tumour specimens received from the Research Repository of Human Brain Tumors and Brain Tissue, UT Southwestern Medical Center and collected according to the IRB-approved protocols. The brain tumour tissue was dissociated mechanically by pushing in between two sterile glass slides and Accutase dissociation system was used to dissociate single cells from the tumour tissue. The cells were then cultured in DMEM F12 supplemented with B27 without Vitamin A, and with EGF (10 ng ml −1 ) and basic fibroblast growth factor (bFGF) (10 ng ml −1 ). A papain dissociation system was used to dissociate tumours and cells were then cultured in Neurobasal medium supplemented with B27 without Vitamin A, and with EGF (10 ng ml −1 ) and bFGF (10 ng ml −1 ). A kinase-inactive EGFR mutant (K721A) was provided by Dr Axel Ullrich. A p5xATF6GL3 construct was provided by Dr Jin Ye. Luciferase assays Cells were plated in 48-well dishes followed by transfection with with pISRE-Luc or IFI27-Luc plasmid [41] using lipofectamine. A dual-luciferase reporter assay system was used according to the instructions of the manufacturer (Promega). Firefly luciferase activity was measured in a luminometer and normalized on the basis of Renilla luciferase activity. Experiments were done in triplicate and three independent experiments were done. RNA interference For transient silencing, we used a pool of siRNA sequences directed against human IRF3, XBP-1, EGFR or control (scrambled) siRNA all obtained from Qiagen. siRNA was performed according to the manufacturer’s protocol using Lipofectamine 2000 reagent (Invitrogen). Experiments were conducted 72 h after siRNA transfection. Antibodies reagents and western blotting Western blot and immunoprecipitation were performed according to standard protocols. EGF was purchased from Peprotech and used at a concentration of 50 ng ml −1 for 15 min unless noted otherwise. In all experiments involving use of EGF, cells were cultured overnight in serum-free DMEM and EGF was added to serum-free DMEM. In such experiments, cells not treated with EGF were also serum starved. Erlotinib was purchased from SellecChem and used at a concentration of 10 μg ml −1 overnight. The PERK inhibitor, GSK 2606414, was purchased from EMD-Millipore and used at a concentration of 1 μM overnight. AEBSF and Thapsigargin were from Sigma and used at a concentration of 300 μM overnight (AEBSF) or 0.5 μM for various time points (Thapsigargin 0.5 μM) as described in figure legends. Temozolomide was from Sigma and used at a concentration of 50 μm. Ruxolinitib (1 μM) and Tofacitinib (300 nM) were from SellecChem and used at a concentration of 1 μM and 300 nM, respectively (overnight). The IFIT1 antibody has been described previously [42] . GAPDH (MAB374), EGFR (06-847) and Shc (06-203) antibodies were from Millipore. pEGFR-1068 (2236), pEGFR-1173 (4407), pEGFR-845 (6963), pERK (4376); pIRF3 (4947), pTBK1 (5483), TBK1 (3504), Lamin B1 (12586), pEIF2α (3398), EIF2α (5324), BiP (3177), IRF7 (4920), TANK (2141), IKKε (2690), pSTAT1 (8062) and STAT1 (9175) antibodies were from Cell Signaling Technology; IRF3, ERK2 (sc-154) pAkt (sc7985), Akt (sc-1619), E-Cadherin (sc-7870), XBP-1 (sc-7160) and actin (sc-47778) were from Santa Cruz Biotechnology. TLR3 antibody was from Abcam (Ab13915). Antibodies were used at a concentration of 1 μg ml −1 . Cetuximab was provided by Imclone and used at a concentration of 100 μg ml −1 overnight unless specified otherwise. Phosphotyrosine (PY20) antibody was from BD Biosciences. Unless specified otherwise, pEGFR refers to phosphoEGFR Y-1068 antibody in this study. Important uncropped western blot images are shown in Supplementary Fig. 18 . ChIP assay U251EGFR, U87EGFR or MDAMB468 cells were plated in 20-cm plates per reaction for ChIP assay (2 × 10 6 cells). The ChIP assay was carried out according to the standard protocols [43] with modifications. Cells were crosslinked by adding formaldehyde (37% (wt/vol)) and incubated for 15 min at room temperature. The cells were scrapped and collected by centrifugation (2,000 g for 5 min at 4 °C) and washed three times with chilled PBS. The cells were lysed by 1 ml immunoprecipitation (IP) buffer (150 mM NaCl, 50 mM Tris-HCl (pH7.5), 5 mM EDTA, 0.5% NP-40 (vol/vol), 1% Triton X-100 (vol/vol)) with protease inhibotors by pipetting up and down. Nuclear pellet was collected by centrtifuging the lysate at 12,000 g for 2 min. The pellet was sonicated until the DNA fragment sizes were 0.5–1 kb. Immunoprecipitation was done by incubating the chromatin fragments with required antibody at 4 °C for 2 h on a rotating rocker. Protein A agarose beads were added the cleared IP samples and incubated for 1 h at 4 °C on a rotating platform. The beads were washed six times with cold IP buffer (1,000 g for 30 s). DNA was isolated by adding 100 μl of Chelex 100 resin slurry (Bio-Rad) and briefly vortexed (10 s) and boiled for 10 min. DNA was precipitated with 2.5 vol of ethanol. The DNA pellet was washed with 70% ethanol for two times. The dried pellet was dissolved in 100 μl Chelex suspension and boiled for 10 min. The supernatant was collected by centrifuging at 12,000 g for 1 min at 4 °C and transferred to a fresh tube and stored at −20 °C for further processing. For PCR, 2 μl of DNA from each reaction was mixed with Platinum Taq DNA polymerase (Invitrogen). For IFI27 promoter the following primers were used: 5′- CATGAGGGGAGAAAgATGTCTGCAGTT -3′ (forward); 5′- CCTCCCTCCCAGTCTTACCCAAAGAAG -3′ (reverse). For IFIT1 promoter, the primers used were: 5′- CCCCCGTCAGCAGGAATTCCGCTAGCTTTA -3′ (forward) and 5′- GCCAGGCTCCTCTGAGATCTGGCT -3′ (reverse). cDNA synthesis and real-time PCR cDNA was prepared from total RNA, using a combination of oligo-dT, random primers, dNTPs and Superscript II (Invitrogen) and Superase.in (RNA inhibitor from Ambion). PCR primers for each gene were obtained from PrimerBank or were designed using Primer3 software, with a melting temperature at 58–60 °C and a resulting product of approximately 100 bp. Each PCR was carried out in triplicate in a 20-μl volume using SYBR Green Master Mix (Applied Biosystems) for 15 min at 95 °C for initial denaturing, followed by 40 cycles of 95 °C for 15 s and 60 °C for 60 s in the ABI prism 7700 sequence Detection system. cDNA prepared from Universal RNA (Stratagene) was used to construct a standard curve for each gene. Two independent experiments were done. Values for each gene were normalized to expression levels of 18S RNA. Primer sequences are available upon request. In vitro binding of IRF3 and EGFR The GST-IRF3 construct has been described previously [44] . GST-IRF3 was immobilized on Glutathione-S-Sepharose beads. PCDNA3-EGFR or empty vectors were subjected to in vitro transcription and translation by using TNT Quick coupled Transcription/Translation kit (Promega) and the reactions were carried out as per the manufacturer’s protocol. Binding reactions were carried out by incubating 20 μl of TNT products of PCDNA3-EGFR-WT or empty vector with 50 μl of GST-IRF3 beads in the presence of NETN buffer (20 mM Tris-HCl, pH 8.0, 100 mM NaCl, 1 mM EDTA, 0.1% Nonidet P-40, 10% glycerol and 2 mM PMSF) for 2 h at 4 °C on a rocking platform, followed by extensive washes. GST alone was used as control. The bound fraction was separated in SDS–PAGE gel and subjected to immunoblotting with EGFR or GST antibody. Cell death/Annexin assay Annexin assay was done by using Annexin-V-FLUOS Staining kit (Roche Applied Science). Cells were cultured in DMEM (10% FBS and Pen/Strep) and serum starved overnight before addition of EGF. Cells (1 × 10 6 ) were plated in six-well plates, infected with adenovirus and treated with EGF (50 ng ml −1 ) or control vehicle. The cells were trypsinized and washed two times with 1 × PBS. The cells were incubated for 25 min at room temperature with propidium iodide and Annexin --FLUOS labelling solution in incubation buffer (supplied by the manufacturer). Annexin- and/or PI-positive cells were detected by flow cytometry. ELISA ELISA kit for quantification of IFI27 and IFN-β levels was purchased from My Biosource and Thermo Scientific, respectively, and used according to the manufacturer’s instructions. Cell fractionation studies Nuclear extracts were made using a kit from Active Motif according to the manufacturer’s instructions. For membrane, cytosolic and nuclear extraction a Qpoteome cell compartment kit from Qiagen and used according to the manufacturer’s instructions. Adenovirus infection Adenovirus-GFP or empty Adenovirus were obtained from Vector Biolabs. An MOI of 10 was used in the experiments. Cells were exposed to adenovirus in the presence or absence of EGF for 24 h followed by immunofluorescence microscopy FACS. For LDL expression experiments, U251MG cells were infected with adenovirus-LDL or empty adenovirus using an MOI of 50. MTT conversion assay An MTT conversion assay was conducted using a kit from Roche Applied Science according to the manufacturer’s protocol. Primary tumours For studies on resected tumour tissue, informed consent was obtained from all subjects. Frozen tissue specimens of human GBMs were obtained according to the IRB-approved protocols at UT Southwestern Medical Center. Resected tumours were initially frozen at −80 °C. Statistical analysis Error bars represent the means±standard deviations of three independent experiments. All data were analysed for significance using GraphPad Prism 5.0 software, where P <0.05 was considered statistically significant. * P ≤0.05, ** P ≤0.01 and *** indicates any P value less than 0.001. How to cite this article: Chakraborty, S. et al . Constitutive and ligand-induced EGFR signalling triggers distinct and mutually exclusive downstream signalling networks. Nat. Commun. 5:5811 doi: 10.1038/ncomms6811 (2014).